A six-carbon 10π-electron aromatic system supported by group 3 metals Aromaticity is a fundamental concept with implications spanning all the chemical sciences. Hückel’s (4n+2)π-electron rule is the standard criterion to determine aromaticity and it applies well to neutral arenes as well as to charged species such as the cyclopentadienyl anion, the cyclooctatetraene dianion and the cycloheptatrienyl cation (tropylium). In the series of all-carbon aromatic compounds, no example of a benzene tetraanion, which is theoretically a 6C, 10π-electron aromatic system, has been reported although heteroatom analogues of such a system, known as ‘electron-rich aromatics’, have been studied in detail for a long time. Here we present the isolation of the first tetraanionic-substituted benzene as a ligand coordinated to group 3 metals. The nature of the substituted benzene tetraanion and the aromaticity of the 6C, 10π-electron system were established by X-ray crystallographic studies, multi-nuclei nuclear magnetic resonance spectroscopy, X-ray absorption spectroscopy and density functional theory calculations. Ever since Michael Faraday isolated benzene in 1825, aromaticity has become one of the most useful chemical concepts [1] . Its scope encompasses not only two-dimensional but also three-dimensional systems, and not only π but also σ orbitals [2] . Oftentimes, however, aromaticity is difficult to define and a host of geometric, energetic and magnetic criteria have been proposed to evaluate its strength in a series of compounds, with disputable success and always stimulating debate. As such, the classic aromaticity of annulene and benzenoid compounds ( Fig. 1 ) is still best predicted and determined by the simple yet powerful Hückel’s (4n+2)π-electron rule [3] . The later discovery of aromaticity in azulene ( Fig. 1 ) reinforced Hückel’s rule as the unfavourable charge separation in this system is overcome by the fulfillment of the (4n+2)π-electron requirement [4] , [5] . The synthesis of a benzene tetraanion (6C, 10π-electron), which is predicted to exhibit aromaticity according to Hückel’s (4n+2)π-electron rule, would expand the series of all-carbon aromatic systems. 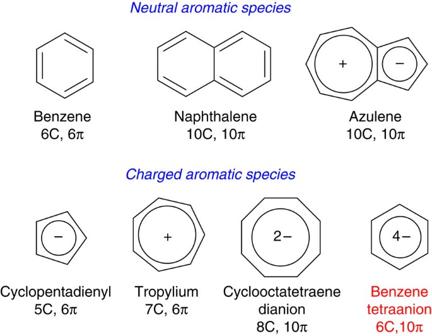Figure 1: Examples of all-carbon aromatic systems. Neutral and charged aromatic systems consisting of five to ten carbon atoms. Figure 1: Examples of all-carbon aromatic systems. Neutral and charged aromatic systems consisting of five to ten carbon atoms. Full size image The hypothetical C 6 H 6 4− was shown computationally [6] to have the largest orbital overlap and the strongest bonds compared with its 10π-electron heteroaromatic analogues [7] . Despite the successful synthesis of S 3 N 3 − (ref. 8 ), P 6 4− (ref. 9 ) and Te 6 2+ (ref. 10 ), however, there are no reports of free C 6 H 6 4− or its derivatives [11] , likely owing to its high negative charge. A successful approach to stabilize benzene polyanions relies on the use of lanthanides and actinides to support the highly reduced benzene ring by coordination. Lappert and co-workers [12] reported the isolation of [(Cp tt 2 La) 2 (μ-η 6 ,η 6 -C 6 H 6 )] (Cp tt =η 5 -1,3- t Bu 2 C 5 H 3 ), which was formulated as an ionic aggregate containing two La(II) ions and the benzene radical monoanion, and [K(18-crown-6)][(Cp′′ 2 Ln)(C 6 H 6 )] (Cp′′=η 5 -1,3-(Me 3 Si) 2 C 5 H 3 ; Ln=La, Ce, Nd), containing Ln(III) and a benzene 1,4-dianion [13] . For actinides, several groups reported that benzene or its derivatives can serve as a bridging ligand between two uranium centers [11] , [14] , [15] , [16] , [17] , [18] , [19] . Magnetic susceptibility measurements, X-ray absorption near edge structure (XANES) spectroscopy and density functional theory (DFT) studies showed that most of these complexes can be described as having a benzene (or a substituted benzene) dianion bridging two U(III) centers [14] , [16] . A [toluene] 4− uranium complex was reported by Liddle and coworkers [11] ; the evidence presented there, however, does not allow an irrefutable interpretation of its electronic structure. We describe for the first time the isolation of tetraanionic, substituted benzenes, which are stabilized by coordination to group 3 metals. Overall, the energetic, structural and magnetic data derived from experiments and theory for complexes incorporating these tetraanionic ligands point to the phenyl ring coordinated to the group 3 metal ions having a 10π-electron aromatic system. The nature of the benzene tetraanion and the aromaticity of the 6C, 10π-electron system are established based on X-ray crystallographic studies, multi-nuclei NMR spectroscopy, X-ray absorption spectroscopy and DFT calculations. Synthesis and structural characterization We have recently reported that 1,1′-ferrocenediamides [20] can support group 3 metal complexes of fused arenes [21] and have since focused on expanding this chemistry to non-fused benzenoid derivatives. Biphenyl was chosen because the two phenyl rings are only weakly conjugated [22] and it has a more accessible reduction potential than benzene ([biphenyl] 0/− at −2.69 V, [benzene] 0/− at −3.42 V and [naphthalene] 0/− at −2.50 V; these values are versus SCE and were calculated according to references) [23] , [24] . Addition of potassium graphite (KC 8 ) to a premixed tetrahydrofuran (THF) solution of (NN fc )YI(THF) 2 ( 1-Y , NN fc =fc(NSi t BuMe 2 ) 2 , fc=1,1′-ferrocenediyl) and biphenyl at −78 °C led to a dark purple solution upon warming to room temperature ( Fig. 2 ). Dark crystals suitable for X-ray crystallography obtained after a standard work up allowed us to determine the molecular structure of the product as [(NN fc )Y] 2 [K(toluene)] 2 (μ-biphenyl) ( 2-Y ) ( Fig. 3a and Supplementary Fig. S94 ). The two yttrium centres are coordinated to opposite sides of the same phenyl ring, while the two potassium ions are coordinated to the other biphenyl ring. Assuming that yttrium is Y(III) and potassium is K(I), the biphenyl ligand carries a 4− charge. XANES spectroscopy studies, commonly used to correlate the electronic structure of metal centres with formal oxidation states [25] , agree with the formulation of yttrium as Y(III) and of iron as Fe(II) in 2-Y (see Supplementary Figs S88—S91 , Supplementary Tables S6, S7 and Supplementary Methods ). 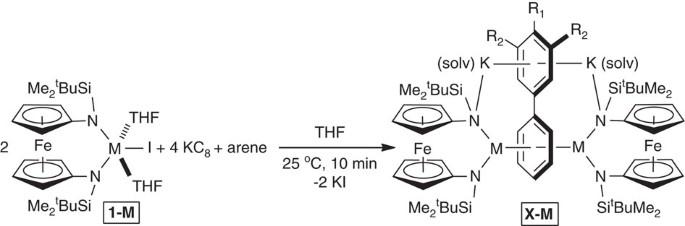Figure 2: Synthesis of quadruply reduced substituted benzene complexes X–M. Solv=THF/Et2O/toluene.X=2, arene=biphenyl,R1=R2=H, M=Sc/Y/La/Lu.X=3, arene=p-terphenyl,R1=phenyl,R2=H,M=Y.X=4, arene=1,3,5-triphenylbenzene,R1=H,R2=phenyl,M=Lu. Figure 2: Synthesis of quadruply reduced substituted benzene complexes X–M. Solv=THF/Et 2 O/toluene. X =2, arene=biphenyl, R 1 =R 2 =H , M =Sc/Y/La/Lu. X =3, arene= p -terphenyl, R 1 =phenyl, R 2 =H, M =Y. X =4, arene=1,3,5-triphenylbenzene, R 1 =H, R 2 =phenyl, M =Lu. 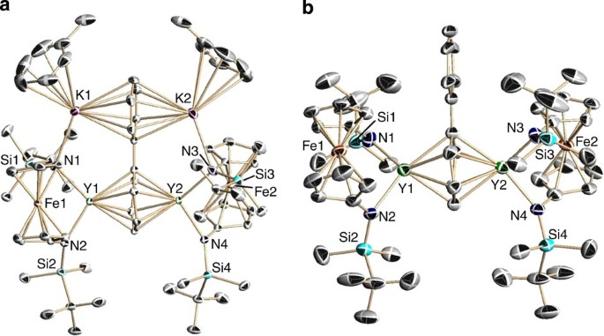Figure 3: Thermal ellipsoid representations. Thermal-ellipsoid (50% probability) representation of2-Y(a) and the anion of2-Y-crown(b). Hydrogen and solvent atoms and disordered counterparts were omitted for clarity. Full size image Figure 3: Thermal ellipsoid representations. Thermal-ellipsoid (50% probability) representation of 2-Y ( a ) and the anion of 2-Y-crown ( b ). Hydrogen and solvent atoms and disordered counterparts were omitted for clarity. Full size image The unusual binding mode of biphenyl in 2-Y with yttrium and potassium coordinated to different rings is of fundamental importance as it suggests that the two aromatic rings are not equivalent. This coordination mode is even maintained in solution. The 1 H NMR spectrum of 2-Y at either 25 °C, −45 °C or −89 °C in THF-d 8 ( Supplementary Figs S13,S16,S19 ) indicated two distinct sets of signals for the phenyl rings. The 1 H NMR pattern for the ring coordinated to the yttrium centres is shifted upfield, while that for the other ring appears in the expected aromatic region (complete assignment of 1 H, 13 C chemical shifts is summarized in Supplementary Table S1 , and compared with other biphenyl dianionic species in Supplementary Table S2 ). In addition, 13 C{ 1 H} NMR spectroscopy showed that the signals for the ortho- and meta-carbon atoms of the ring coordinated to yttrium are triplets owing to coupling to yttrium; [26] the para and ipso carbon atoms, being the farthest from the yttrium ions, are not coupled to them and appear as singlets. These findings are consistent with the fact that only one of the two phenyl rings is coordinated to both yttrium ions in solution. It is worth mentioning that previously reported lanthanide arene complexes usually exhibit fluxional behaviour in solution even when their solid-state structures indicate that the two metal centres coordinate to different phenyl rings, as reported for doubly reduced biphenyl yttrium complexes [27] . In our case, no fluxional behaviour was observed in solution. In addition, the isolation of the 18-crown-6 version of 2-Y , [K(18-crown-6)(THF) 2 ] 2 [[(NN fc )Y] 2 (μ-biphenyl)] ( 2-Y-crown ), indicated that the coordination of potassium ions to the biphenyl ligand is not required to maintain the rigid structure. The solid-state molecular structure of 2-Y-crown ( Fig. 3b and Supplementary Fig. S97 ) showed the presence of separated ion pairs of [[(NN fc )Y] 2 (μ-biphenyl)] 2− and two [K(18-crown-6)(THF) 2 ] + . The chemical shifts of the resonances in the 1 H and 13 C NMR spectra (THF-d 8 , 25 and −45 °C, Supplementary Figs S42—S47 ) of 2-Y-crown were only slightly different from those of the corresponding resonances documented for 2-Y , suggesting that 2-Y is likely a separated ion pair in THF-d 8 solution as well. We also observed that 2-Y formed exclusively even when sub-stoichiometric amounts of KC 8 were used, suggesting that the quadruply reduced biphenyl in 2-Y is more stable than a doubly reduced yttrium biphenyl complex [27] . In addition, a comproportionation reaction between 1-Y and 2-Y did not occur to give a doubly reduced biphenyl complex. Attempts were made to oxidize selectively the quadruply reduced arene to a doubly reduced species but they failed (see Supplementary Methods for details). The synthesis of 2-Y is not an isolated instance: other group 3 metals, namely, scandium, lanthanum and lutetium, form 2-Sc , 2-La and 2-Lu , respectively, following a synthetic protocol analogous to that for 2-Y ( Fig. 2 ). The 1 H and 13 C NMR spectra ( Supplementary Figs S26—S34 ) and solid-state molecular structures of these complexes ( Supplementary Figs S95,S96 ) reflect their similarity to 2-Y ( Supplementary Table S1,S3 ). The generality of this reduction reaction also applies to other non-fused arenes. When using p -terphenyl instead of biphenyl, [(NN fc )Y] 2 [K(THF) 2 ] 2 [μ-(p-terphenyl)] ( 3-Y ) was obtained ( Fig. 2 ). The solid-state molecular structure ( Supplementary Fig. S98 ) and solution 1 H and 13 C NMR spectra of 3-Y ( Supplementary Figs S35—S37 ) showed that one of the end rings was bridging the two yttrium centres ( Supplementary Table S1 ). 1,3,5-triphenylbenzene was also examined in the reaction with 1-Lu ( Fig. 2 ). Compound 4-Lu is analogous to 2-Lu , with one end ring coordinating to the two lutetium fragments ( Supplementary Fig. S99 ). The confirmed features of the bridging arenes, namely quadruple reduction, rigid coordination mode and the relative stability, over the doubly reduced complexes brought up the fundamental question of whether these species could be considered examples of a 6C, 10π-electron aromatic system according to Hückel’s (4n+2)π-electron rule. Structurally, an ideal aromatic system exhibits similar bond lengths and planarity of the atoms involved in π conjugation. In C 6 H 6 4− , because the two e 2u vacant orbitals (π 4 and π 5 , Fig. 5d) of benzene are filled, there is one net π bonding orbital. Compounds 2-M ( M =Y, Sc and Lu), 2-Y-crown , 3-Y and 4-Lu exhibit similar C–C distances of the coordinated phenyl ring (average of 1.46 Å for 2-Y and 1.47 Å for 2-Y-crown in Fig. 4 , see Supplementary Table S3 for other complexes) that are significantly different and longer than those in neutral biphenyl (1.39–1.42 Å for intra-ring and 1.48 Å for inter-ring distances) [28] or the non-coordinated ring (1.41 Å for 2-Y and 1.38 Å for 2-Y-crown ). The average distance of 1.47 Å ( 2-Y-crown ) is the longest reported average C–C distance within a single benzene ring, and close to the value calculated for the elusive C 6 H 6 4− (1.507 Å; this value was found to be consistent with the presence of aromatic character; the calculated values for the electron-rich heteroaromatics were found to be higher than experimental values) [6] . The fact that the C–C distances within the ring coordinated to yttrium of 2-Y (1.486, 1.477 and 1.422 Å) or 2-Y-crown (1.496, 1.489 and 1.441 Å) are slightly different and that the values for the C ipso –C ipso distances and the C–C bonds in the non-coordinating ring vary may be explained by the localized molecular orbital model and corresponding drawing of resonance canonical structures [6] or by taking into account small contributions from other resonance structures (see below). All six C–C–C angles in the coordinated phenyl ring are close to 120°, which is the calculated value for the hypothetical C 6 H 6 4− with D 6h symmetry [6] . It was noticed that the phenyl ring coordinated to yttrium exhibited a small torsion angle (defined by the atoms C 24 , C 25 , C 25 * and C 24 *) of 11.4° ( 2-Y ) or 12.4° ( 2-Y-crown ). This angle was slightly larger in 2-Sc (20.4°) and 2-Lu (19.7°). These distortions may be caused by a second-order Jahn–Teller effect that is well documented for reduced arenes [29] . 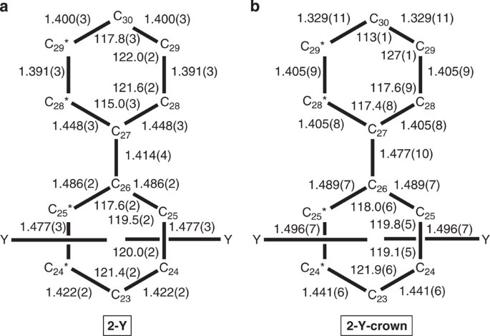Figure 4: Metrical parameters. Metrical parameters for the biphenyl ligand in2-Y(a) and2-Y-crown(b). Distances are in Å and angles in °, with the errors showed in parentheses. For2-Y-crown, C29and C30are disordered, therefore, the C29–C30distance and the C28–C29–C30and C29–C30–C29* angles are not reliable. Figure 4: Metrical parameters. Metrical parameters for the biphenyl ligand in 2-Y ( a ) and 2-Y-crown ( b ). Distances are in Å and angles in °, with the errors showed in parentheses. For 2-Y-crown , C 29 and C 30 are disordered, therefore, the C 29 –C 30 distance and the C 28 –C 29 –C 30 and C 29 –C 30 –C 29 * angles are not reliable. Full size image DFT calculations DFT calculations showed that optimized structures for models of 2-Y / 2-Y-crown are in excellent agreement with the experimental findings, with average C–C distances of 1.472–1.479 Å for the coordinated phenyl ring ( Supplementary Tables S8,S9 ). The ground state was found to be a singlet, with no unpaired electrons on the yttrium ions and an iron(II) electronic configuration, in agreement with the oxidation states derived from the XANES measurements. As depicted in Fig. 5 , inspection of the Kohn–Sham frontier molecular orbitals confirms the presence of a benzene unit reduced by four electrons. Indeed, the highest occupied molecular orbital (HOMO) and HOMO-1 clearly result from the population of the two e 2u vacant orbitals (π 4 and π 5 ) of the benzene motif. The computed natural bond orbital charges ( Supplementary Tables S8,S9 ) for the coordinated benzene ring (−1.90 to −1.95) and the uncoordinated phenyl group (−0.26 to −0.27) are significantly different. This confirms the experimental observation that negative charges are mainly localized on the coordinated phenyl ring, while the uncoordinated phenyl ring acts only as an electron withdrawing group. Importantly, the putative complex 5-Y 2− , in which each yttrium ion is coordinated to a different benzene ring, could also be investigated computationally for comparison. HOMO and HOMO-1 of 5-Y 2− ( Fig. 5f ) establish that only one e 2u vacant orbital (π 5 ) on each ring is occupied, leaving two anti-aromatic 8π-electron ligands. The charge distribution in 5-Y 2− is symmetrical, each ring bearing a charge of −1.05 ( Supplementary Table S13 ). More interestingly, the anti-aromatic character of 5-Y 2− is attested by the 20.7 kcal mol −1 energy gap with respect to its more stable aromatic isomer 2-Y 2− , in agreement with the absence of fluxionality established experimentally (see Supplementary Methods for details). 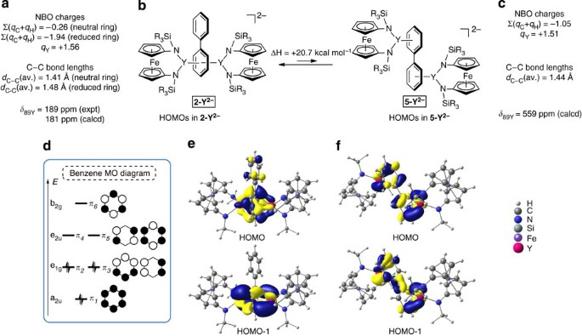Figure 5: DFT calculations on the electronic structure, energetic and magnetic properties of anions 2-Y2−(C2symmetry) and 5-Y2−(S2symmetry). (a) Calculated natural bond orbital (NBO) charges for the tetraanionic biphenyl ligand and yttrium, C–C distances for the tetraanionic biphenyl ligand and comparison between the experimental and calculated89Y chemical shift for2-Y2−. (b) Equilibrium between the tetraanionic-substituted benzene complex (2-Y2−) and a hypothetical tetraanionic biphenyl complex, in which each ring coordinated to yttrium is dianionic (5-Y2−). (c) Calculated NBO charges for the tetraanionic biphenyl ligand and yttrium, C–C distances for the tetraanionic biphenyl ligand and calculated89Y chemical shift for5-Y2−. (d) Frontier molecular orbitals in free benzene. (e) HOMO and HOMO-1 Kohn–Sham orbitals of2-Y2−. (f) HOMO and HOMO-1 Kohn–Sham orbitals of5-Y2−. Figure 5: DFT calculations on the electronic structure, energetic and magnetic properties of anions 2-Y 2− (C 2 symmetry) and 5-Y 2− (S 2 symmetry). ( a ) Calculated natural bond orbital (NBO) charges for the tetraanionic biphenyl ligand and yttrium, C–C distances for the tetraanionic biphenyl ligand and comparison between the experimental and calculated 89 Y chemical shift for 2-Y 2 − . ( b ) Equilibrium between the tetraanionic-substituted benzene complex ( 2-Y 2 − ) and a hypothetical tetraanionic biphenyl complex, in which each ring coordinated to yttrium is dianionic ( 5-Y 2− ). ( c ) Calculated NBO charges for the tetraanionic biphenyl ligand and yttrium, C–C distances for the tetraanionic biphenyl ligand and calculated 89 Y chemical shift for 5-Y 2 − . ( d ) Frontier molecular orbitals in free benzene. ( e ) HOMO and HOMO-1 Kohn–Sham orbitals of 2-Y 2 − . ( f ) HOMO and HOMO-1 Kohn–Sham orbitals of 5-Y 2 − . Full size image 89 Y NMR spectroscopy Among experimental methods to determine aromaticity, chemical shifts of NMR active nuclei at specific positions are especially useful [30] , [31] . Fortunately, among group 3 metals, yttrium has a 100% naturally abundant isotope with spin ½. Though 89 Y suffers from low sensitivity (1/133 of that of 13 C) and requires prolonged relaxation times in solution (typically over 300 s) [32] , we obtained 89 Y chemical shifts for a series of compounds ( Supplementary Table S5 ) containing different groups, including halide, alkyl and the aromatic anion Cp: 1-Y , (NN fc )Y(CH 2 Ph)(THF) 2 ( Y-Bn ) and (NN fc )Y(Cp)(THF) ( Y-Cp ) together with 2-Y and 3-Y . We found that the value (in ppm) of the 89 Y chemical shift decreased in the series: Y-Bn (+436), 1-Y (+370), 3-Y (+213), 2-Y (+189), Y-Cp (+69). This result confirms significant aromatic ring current effects of the phenyl ring coordinating to yttrium in 2-Y and 3-Y as 89 Y chemical shifts in 2-Y and 3-Y are different from Y-Bn and 1-Y , but closer to Y-Cp , which contains the aromatic ligand Cp. The 89 Y downfield shifts of 2-Y and 3-Y compared with that of Y-Cp are expected because the net π bond order in the non-coordinating phenyl ring is only 1. Computational studies of NMR parameters have proved successful in the past for organometallic complexes, even for heavy atoms such as 89 Y (ref. 33 ). The calculated 89 Y chemical shifts (in ppm) for Y-Bn (+451), 1-Y (+350), 3-Y (+212), 2-Y (+181) and Y-Cp (+77) are in excellent agreement with the experimental values and allowed us to compute the 89 Y chemical shift of the anti-aromatic isomer [5-Y] 2− to be +559 ppm. This change ongoing from 2-Y to 5-Y corroborates the structural, electronic and energetic data discussed above and points to the aromatic character of 2-Y . The fact that 2-Y and 3-Y have similar chemical shifts that are greatly different from those of 1-Y and Y-Cp supports the assignment of a 6C, 10π-electron aromatic system for the yttrium-coordinated phenyl ring. Altogether, these results support the description of 2-Y (and 3-Y ) as coordinated 6C, 10π-electron tetraanionic benzene ligands. The correct match of the trend of 89 Y chemical shifts found by us also demonstrates the potential of utilizing 89 Y NMR spectroscopy in characterizing aromatic currents in highly reduced π-conjugated systems. The isolation of tetraanionic, substituted benzenes was possible because of their coordination to group 3 metals. Based on experimental and computational data, we propose that the phenyl ring coordinated to the group 3 metal ions has a 10π-electron aromatic system. 89 Y NMR spectroscopy and DFT calculations of the tetranionic biphenyl metal complexes were instrumental in understanding the proposed electronic structure. In addition to the group 3 metals, the phenyl substituents of the reduced benzene ring also have a stabilizing influence on the four-electron reduction state of the arene ligands. In addition to the structures described above, we also considered the possibility of two limit Lewis structures that may describe the distribution of the additional four electrons in the reduced arene ligands: a 7C, 10π-electron structure, in which a trianionic benzyl fragment is substituted by a pentadienyl anion, and a 6C, 10π-electron structure, as discussed above, in which the four highest energy electrons are located on a single benzene ring and the phenyl substituent remains neutral ( Fig. 6 ). The two limit structures differ by the amount of electronic density located on the phenyl substituent. Model complexes [6-Y] 2− and [7-Y] − illustrate each Lewis structure, respectively, and their geometrical and electronic characteristics were investigated computationally ( Fig. 6 and Supplementary Fig. S102 ). While [6-Y] 2− has frontier molecular orbitals, bond lengths and charge distributions similar to the [2-Y] 2− model, the computational data gathered for complex [7-Y] − strongly differ from those of [2-Y] 2− . Indeed, the exocyclic C=C bond in 7-Y is much shorter than in [2-Y] 2− (calculated values of 1.37 versus 1.45 Å) and HOMO-1 is mostly located on the exocyclic C=C bond, leaving the π 5 orbital of the benzene ring vacant ( Supplementary Fig. S102 ). In addition, the 89 Y chemical shift computed for [6-Y] 2− (117 ppm) is more shielded than the shift calculated for [7-Y] − (311 ppm) and closer to 2-Y (181 ppm) ( Supplementary Table S11 ). 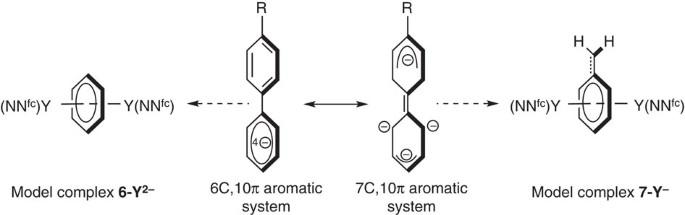Figure 6: Lewis structures. Possible Lewis structures for the tetraanionic ligands in2-Y,2-Y-crownand3-Y, and drawing of model complexes[6-Y]2−and[7-Y]−. Figure 6: Lewis structures. Possible Lewis structures for the tetraanionic ligands in 2-Y , 2-Y-crown and 3-Y , and drawing of model complexes [6-Y] 2− and [7-Y] − . Full size image An interesting analogy between the present work and two reports by Pierrefixe and Bickelhaupt [34] , [35] can be made: in those reports, it was shown that the regular structure of aromatic cores with equivalent partial double bonds (6C, 6π and 10C, 10π-electron systems) stems from the σ skeleton and not from the π-electrons. Naphthalene prefers localized double bonds, a behaviour that can be understood from the fact that the π overlap increases as the C–C bond becomes shorter and reaches its maximum at 0 Å. On the other hand, σ-bond overlap achieves its optimum around 1.5 Å for all C–C bonds. Thus, the σ electrons are responsible for the highly symmetric structure. From this work, it follows that reducing the aromatic 6C, 6π-electron system towards the 6C, 10π-electron system weakens the bond localizing tendency of the π electrons because e* type orbitals are being filled. Pierrefixe and Bickelhaupt illustrated that effect by going from benzene to planar cyclohexane (6C, 12π). Although the benzene tetraanion described by us is thermodynamically less stable and more reactive (it has to be stabilized through coordination) than benzene, according to the structural considerations described by Pierrefixe and Bickelhaupt, it shows higher aromaticity than benzene. The benzene tetraanionic fragments reported here expand the series of all-carbon aromatic systems. Although C 6 H 6 4− in its free form may prove elusive to synthetic chemists, the examples reported here further our understanding of aromaticity and of the ability of metal complexes to stabilize reactive fragments. General considerations All experiments were performed under a dry nitrogen atmosphere using standard Schlenk techniques or an MBraun inert-gas glove box unless otherwise specified. All newly synthesized compounds were characterized by 1 H, 13 C and 89 Y (if applicable) NMR spectroscopy, single crystal X-ray diffraction and confirmed by elemental analysis for purity. Reactions were monitored by 1 H NMR spectroscopy. Fe K-edge (7,112 eV) and Y K-edge (17,038 eV) X-ray absorption measurements were conducted on the bending magnet beamline of the Materials Research Collaborative Access Team (MRCAT, 10-BM) at the Advanced Photon Source (APS), Argonne National Laboratory. Synthesis of [(NN fc )M] 2 [K(solvent)] 2 (μ-biphenyl) (2-M) The procedure for synthesizing arene-bridged complexes is similar and only that for 2-Y is described below. Synthesis of 2-Y 0.4680, g of 1-Y (0.583 mmol) and 0.0450, g of biphenyl (0.292 mmol) were weighed in the same vial and dissolved in 8 ml of THF. The solution was placed in a dry ice/acetone bath for 10 min before the addition of 0.1890, g KC 8 (1.40 mmol). After the addition, the mixture was taken out from the dry ice/acetone bath and stirred at 25 °C for 10 min. Right after the addition, the solution colour changed from bright yellow to dark. The solution was then filtered through Celite adding a small amount of Et 2 O to help the transfer. The volatiles were removed under reduced pressure. The remaining dark solids were dispersed in Et 2 O, transferred to a vial and stored at −35 °C for 1 day. Black microcrystals were collected on a medium frit. Yield: 0.2420, g, 57.6%. Single crystals suitable for X-ray crystallography were obtained from a THF solution layered with toluene and hexanes with a molecular formula of [(NN fc )Y] 2 [K(toluene)] 2 (μ-biphenyl). 1 H, 13 C, 89 Y and HMBC NMR spectra of all newly synthesized compounds and relevant reaction aliquots are included as Supplementary Figs S1—S87 . Molecular structures are included as Supplementary Figs S92—S101. For complete experimental details and characterization of new compounds, see Supplementary Methods . Computational details DFT calculations were carried out using the program Gaussian09 and employed the B3LYP hybrid density functional to optimize the equilibrium molecular structure of the model complexes. Calculations were first run on various models for 2-Y to determine whether the alkyl substituents can be replaced by hydrogen atoms ( Supplementary Table S8 ). In all other model structures, the alkyl substituents on the silicon atoms were replaced by hydrogen atoms. The yttrium atoms were represented by the relativistic effective core potential from the Stuttgart group and the associated basis sets. 6-31+G* basis sets were used for carbon, hydrogen, nitrogen, oxygen and silicon for all models although calculations with other basis sets were also carried out. The LANL2DZ effective core potential and valence double zeta basis set was used for iron and iodine. For DFT calculation details, see Supplementary Figs S102—S107 , Supplementary Tables S8—S28 and Supplementary Methods . 89 Y NMR spectroscopy details All 89 Y NMR spectra were measured on a Bruker AV600 spectrometer with a 5-mm broadband probe with z-gradient at frequency 29.40 MHz using C 4 D 8 O as a solvent. Two data collection settings were used: zg30 pulse program with d1=59 s and ns=1024 or more; zg90 pulse program with d1=300 s and ns=160 or more. 89 Y chemical shifts were referenced to YCl 3 in D 2 O used as an external standard (0 ppm) at 25 °C. Y-Bn, 1-Y, YBn 3 , Y-Cp and Cp 3 Y(THF) were measured at 25 °C; 2-Y and 3-Y were measured between −40 to −50 °C to avoid decomposition during data collection. A temperature dependence study was carried out for 1-Y and Y-Cp . 1-Y : 25 °C, +369.6 ppm; −44 °C, +369.9 ppm Y-Cp : 25 °C, +68.8 ppm; −44 °C, +69.6 ppm. The study showed a small temperature dependence of 89 Y chemical shifts. Accession codes: The X-ray crystallographic coordinates for structures reported in this Article have been deposited at the Cambridge Crystallographic Data Centre (CCDC), under deposition number CCDC 916586—916595. These data can be obtained free of charge from The Cambridge Crystallographic Data Centre via www.ccdc.cam.ac.uk/data_request/cif . How to cite this article: Huang, W. et al. A six-carbon 10π-electron aromatic system supported by group 3 metals. Nat. Commun. 4:1448 doi: 10.1038/ncomms2473 (2013).